Injectable bioadhesive hydrogels with innate antibacterial properties Surgical site infections cause significant postoperative morbidity and increased healthcare costs. Bioadhesives used to fill surgical voids and support wound healing are typically devoid of antibacterial activity. Here we report novel syringe-injectable bioadhesive hydrogels with inherent antibacterial properties prepared from mixing polydextran aldehyde and branched polyethylenimine. These adhesives kill both Gram-negative and Gram-positive bacteria, while sparing human erythrocytes. An optimal composition of 2.5 wt% oxidized dextran and 6.9 wt% polyethylenimine sets within seconds forming a mechanically rigid (~\n1,700 Pa) gel offering a maximum adhesive stress of ~\n2.8 kPa. A murine infection model showed that the adhesive is capable of killing Streptococcus pyogenes introduced subcutaneously at the bioadhesive’s surface, with minimal inflammatory response. The adhesive was also effective in a cecal ligation and puncture model, preventing sepsis and significantly improving survival. These bioadhesives represent novel, inherently antibacterial materials for wound-filling applications. Surgical site infections can result in prolonged wound healing, wound dehiscence, abscess formation and, in severe cases, sepsis. These infections represent a significant clinical burden in that patients are typically readmitted, often into intensive care units and are at higher risk of further complications [1] . Incision sites and dead spaces are fertile infection locales, especially those in non-vascularized areas where the immune system has difficulty in detecting the infection, as well as those in areas of high adipose content that are nutrient rich for bacteria [2] . Materials that can be applied to damaged tissue during surgery that thwart infection would be clinically useful. Bioadhesive materials adhere to tissue by forming chemical cross-links [3] , [4] , [5] , [6] , [7] , or by mechanically fixing [8] themselves to components of the extracellular matrix (ECM). Although this mechanical property enables many potential applications, their use as wound sealants and void fillers has reached the clinic. For example, the fibrin-based adhesive, Tisseel (Baxter), takes advantage of endogenous Factor XIII-transglutaminase to cross-link fibrin to itself, as well as to components of the ECM [9] , [10] . As with any material introduced to a surgical site, infection is of concern. For patients undergoing medical procedures, surgical site infections are the most common type of infection encountered in the nosocomial environment [11] . For wound-filling applications, using a material that is adherent affords a well-integrated material–tissue interface that limits the potential formation of dead space micro-pockets that could foster infection. Thus, developing bioadhesives that can integrate well with tissue and also kill bacteria should significantly decrease the occurrence of surgical site infections. Antibacterial properties can be imparted to a material by doping in an exogenous antibiotic for eventual release [12] . In these systems, the active agent is released from the polymer matrix over time and the material’s antibiotic activity is eventually exhausted with the remaining matrix being left inactive. One way to overcome this limitation is to prepare materials that are themselves antibiotic. Although not strictly developed for biomedical applications, antibacterial properties have been endeared to glasses [13] , fabrics [14] , [15] and metals [16] , [17] by covalently attaching cationic functional groups to their surfaces. The mechanisms responsible for the activity of positively charged surfaces are still debated; however, they typically involve bacterial cell depolarization and/or membrane disruption leading to cell lysis [18] . We envisioned that the cationic functionality enjoyed by the hard surfaces discussed above could be imbibed into the nanostructural network of an injectable soft material adhesive. 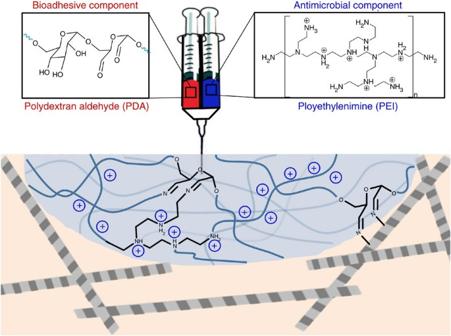Figure 1: Design of injectable bioadhesive hydrogels with antibacterial activity. The precursor components of the adhesive, PDA and PEI, define the material’s bioadhesive and antibacterial properties, respectively. Figure 1 shows the design of a two component adhesive that can be delivered from a dual barrel syringe. Polydextran aldehyde (PDA) serves as the adhesive component capable of reacting with endogenous amines of the ECM through imine bond formation, defining the adhesive properties of the material [19] . The second component, branched polyethylenimine (PEI), serves to cross-link the dextran aldehyde, again through imine bond formation, defining the cohesive nature of the material. PEI and its derivatives have been extensively used in drug and gene delivery, the formulation of nanoparticles and as surface coatings [20] . PEI contains a large fraction of protonated amines at physiological pH that can bind to negatively charged components of bacterial cell surfaces ultimately resulting in a number of events, including cell depolarization, cell wall/membrane disruption and cell lysis. For example, when soluble PEI is added to cultures of Gram-negative bacteria, it binds to components of and permeabilizes their outer membranes making the bacteria more susceptible to exogenous antibiotics [21] . Soluble branched PEI is also known to be antibacterial on its own having minimum inhibitory concentration values of 0.09 mg ml −1 for Escherichia coli and 0.1 mg ml −1 for Staphylococcus aureus [22] . When immobilized to surfaces, N-alkylated PEI is capable of avidly killing bacteria on contact via membrane disruption while sparing mammalian cells [13] . Although there are reports of PEI-based cytotoxicity [23] , chemical functionalization and/or immobilizing the polymer to a material can greatly diminish this undesirable trait [13] , [20] , [24] , [25] . Figure 1: Design of injectable bioadhesive hydrogels with antibacterial activity. The precursor components of the adhesive, PDA and PEI, define the material’s bioadhesive and antibacterial properties, respectively. Full size image Herein we describe the design, synthesis and assessment of a bioadhesive whose innate antibacterial, mechanical and biological properties suggest its use as a general dead space filler for wound closure to prevent bacterial growth and infection. Important to our application, employing PEI as a cross-linker imbibes positive charge to the adhesive’s polymeric network and renders it a potent antibacterial. We systematically study the influence of PEI content on the material’s mechanical and biological properties affording an optimal formulation that sets at a rate conducive to surgical delivery, is mechanically stiff and adheres to tissue. The adhesive can kill both Gram-negative and Gram-positive bacteria, while being cyto- and bio-compatible as assessed in vitro and in vivo , respectively. Mechanical characterization of bioadhesive formulations Four different material compositions were examined, with the PDA component held constant at 2.5 wt%, while the concentration of PEI was varied from 3.5 to 10.3 wt%. In Table 1 , the variable concentrations of PEI are listed with the corresponding RNH 2 /RCHO ratios, along with each formulation’s average gelation time ( t gel ), storage modulus (G′) and maximum adhesive stress value. The preparation of PDA and branched PEI, as well as the determination of gelation times for the different formulations of bioadhesive, are detailed in the Supplementary Methods . The RNH 2 /RCHO ratio serves as a convenient parameter to rationalize material performance and is defined by the starting concentrations of PEI and PDA, respectively, before the components are mixed. Table 1 shows that as the RNH 2 /RCHO ratio increases, the adhesive forms more quickly on mixing of the two components. This is due to the greater number of primary amines available for reaction at higher ratios. We have found that a gelation time of 5–15 s is optimal for syringe delivery for in vivo applications, allowing sufficient time for tissue manipulation after the adhesive has been administered. The mechanical stiffness (G′) of each formulation was measured on pre-formed gels by oscillatory rheology. As the RNH 2 /RCHO ratio increases, the stiffness of the material also increases from ~\n600 to ~\n4,500 Pa. This suggests that formulations having a greater number of primary amines can form more imine cross-links with available aldehydes, thus increasing the stiffness of the material. Lastly, the adhesive nature of the material was studied by performing a lap-shear analysis during uniaxial loading of the material adhered between two strips of porcine epidermis as defined by the American Society for Testing and Materials (ASTM) standard protocol F2255. Table 1 shows that the maximum adhesive stress is invariant with the RNH 2 /RCHO ratio, being around 2 kPa, which is on the order of that observed for clinically used fibrin glue as measured in our lab ( Supplementary Fig. 1 ). We observed that the mode of bond failure for our material was largely cohesive in nature, indicating that cross-links within the bulk material fail first rather than interactions that define the material-tissue interface. This suggests that the porcine ECM contains a relatively large concentration of amines or other functional groups that can react with the material as it cures. This data, taken together, suggests that adhesives formed at RNH 2 /RCHO ratios of 3–4 provide optimal curing times and mechanical properties that are suitable for bioadhesive applications. Table 1 Mechanical properties of respective formulations. Full size table In vitro antibacterial properties and mechanism of action We next examined the in vitro antibacterial activity of the bioadhesive’s surface towards model Gram-negative and -positive bacteria, E. coli and S. aureus , respectively. 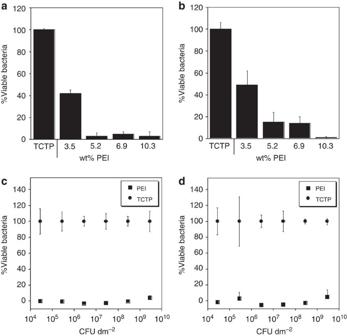Figure 2: Antibacterial surface properties of adhesive hydrogels. PDA cross-linked with variable concentrations of PEI were challenged with 104CFU ml−1(a)E. colior (b)S. aureus, for 24 h (n=3). TCTP alone ([cirf ]) and PDA cross-linked with 6.9 wt% PEI (▪) surfaces challenged with increasing concentrations of (c)E. colior (d)S. aureus(n=3; error bars, s.d.). Figure 2a,b show the results from an assay in which the surface of adhesives prepared with varying amounts of PEI were challenged with 10 4 CFU ml −1 of bacteria. Bacterial viability was assessed 24 h after inoculating the surfaces. Tissue culture treated polystyrene (TCTP) was used as a control surface. The data show that as the weight percent of PEI increases in the formulation, the antibacterial activity of the adhesive’s surface increases for both E. coli and S. aureus . For example, at 3.5 wt% PEI the surfaces are moderately active. However, if the weight percent is increased to ≥5.2 the surfaces become extremely active. This PEI concentration-dependent behaviour suggests that the protonated amine content of the adhesive directly influences its antibacterial activity. Although the degree of protonation of the gel’s PEI component is not known, literature suggests that up to 50% of the amines could be in the protonated state at physiological pH [26] . It should be mentioned that PDA has been reported to display antibacterial activity [27] with minimum inhibitory concentration towards E.coli of 32 mg ml −1 and S. aureus of 4 mg ml −1 . Thus, we cannot rule out that PDA may also contribute to the adhesive’s antibacterial properties. The activity of the adhesive was further studied by challenging its surface with an increasing number of colony-forming units (CFUs) of bacteria. Figure 2c,d show percent viable bacteria as a function of increasing CFU for an adhesive prepared from 6.9 wt% PEI. The data clearly show that this adhesive’s surface is extremely active against both E. coli and S. aureus even at 10 9 CFU dm −2 . This number of bacteria is about ten million times greater than would be expected even for a contaminated operating theatre [28] . In contrast, when the same number of bacteria was introduced to the TCTP control surface, uninhibited growth was observed. Figure 2: Antibacterial surface properties of adhesive hydrogels. PDA cross-linked with variable concentrations of PEI were challenged with 10 4 CFU ml −1 ( a ) E. coli or ( b ) S. aureus , for 24 h ( n =3). TCTP alone ([cirf ]) and PDA cross-linked with 6.9 wt% PEI (▪) surfaces challenged with increasing concentrations of ( c ) E. coli or ( d ) S. aureus ( n =3; error bars, s.d.). Full size image Although not definitively proven, the data in Fig. 2 suggests a contact-dependent mechanism of action that involves bacterial engagement of the adhesive’s surface. The mechanism was further probed by performing a competitive cytotoxicity assay. Here, pre-formed slab agar gels were employed that had a cylindrical portion of their agar removed. The resulting hole was filled with 6.9 wt% PEI adhesive, resulting in a bulk surface that contained a circular area of adhesive surrounded by agar. This surface was exposed to trypic soy broth containing 10 8 CFU ml −1 E. coli and incubated for 24 h at 37 °C. 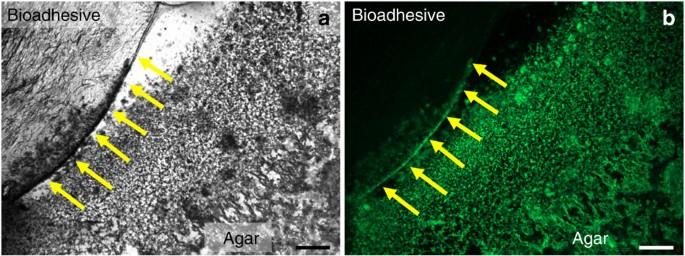Figure 3:E. coliviability on antibacterial bioadhesive surfaces. E. coliviability was monitored after 24 h of incubation on neighbouring bioadhesive and agar surfaces (n=3). Representative images shown. (a) The bright-field image defines the boundary between the bioadhesive and agar materials. (b) Viable bacteria fluoresce green only on the agar surface (scale bars, 0.5 mm). Figure 3 shows bright-field and confocal micrographs of a quadrant of the adhesive surrounded by agar. The interface between the adhesive and agar is evident in both the bright-field and confocal micrographs. Viable bacterias were stained with Syto9, a green DNA fluorescent probe. The lack of green fluorescence observed on the bioadhesive indicates that bacteria were incapable of adhering and proliferating on the surface of the adhesive. However, the pronounced fluorescence on the neighbouring agar surface demonstrates that E. coli maintains its ability to attach and proliferate when given a biocompatible surface. The data in Figs 2 and 3 suggests that bacteria must engage the material to be killed. However, it is possible that free PEI could be leaching from the adhesive and exerting action. This possibility was tested by preparing 6.9 wt% PEI adhesive gels within separate transwell cell culture inserts. These inserts were then placed in culture wells above, and spatially separated from lawns of bacteria proliferating on the polystyrene surface below. If PEI is capable of leaching from the adhesive into the culture media, bacterial death should result. After a 24-h incubation, no cell death was observed for both E. coli and S. aureus cultures, indicating that the PEI had not leached from the adhesive ( Supplementary Fig. 2 ). In contrast, when soluble PEI alone was added to the insert, bacteria proliferation was greatly inhibited. Taken together, the data indicate that the bioadhesive, is itself, inherently antibacterial. Figure 3: E. coli viability on antibacterial bioadhesive surfaces. E. coli viability was monitored after 24 h of incubation on neighbouring bioadhesive and agar surfaces ( n =3). Representative images shown. ( a ) The bright-field image defines the boundary between the bioadhesive and agar materials. ( b ) Viable bacteria fluoresce green only on the agar surface (scale bars, 0.5 mm). Full size image We next studied the cytotoxic selectivity of the adhesive’s surface with respect to prokaryotic versus eukaryotic cells. Previous studies have shown that cationic surfaces can disrupt the structural integrity of bacterial cell surfaces leading to lysis and/or cellular depolarization [18] . The surface of bacteria are negatively charged, primarily a result of negatively charged lipids comprising their membranes as well as the electronegative macromolecules that decorate their surfaces such as lipopolysaccharide and teichoic acid, present in Gram-negative and -positive bacteria, respectively [29] . Unlike prokaryotic cells, eukaryotic cells, such as human erythrocytes, are rich in zwitterionic lipids and sterols, such as cholesterol and ergosterol, which have been shown to stabilize their membranes [30] , [31] . Although the differences in membrane architecture between prokaryotic bacteria and eukaryotic cells are numerous and significant, there remains enough similarity that our bioadhesive might not differentiate between bacteria and mammalian cells. 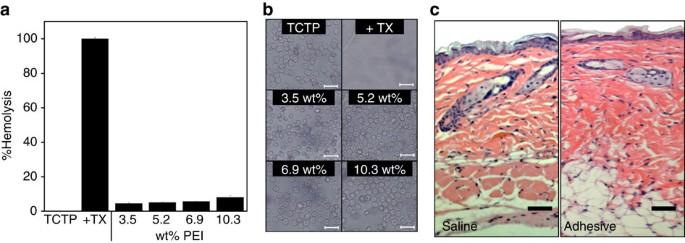Figure 4:In vitroandin vivobiocompatibility of adhesive. (a) Haemolytic activity of adhesives as a function of PEI wt% along with the control TCTP surface with and without Triton-X (TX) (n=3; error bars, s.d.). (b) Phase-contrast images of hRBCs plated on adhesives of varying PEI wt% or on the control TCTP surface with and without Triton-X (TX) (scale bars, 20 μm). (c) Histological examination of tissue at the injection site for the sham saline injection and the adhesive. No necrosis is evident in either sample and minimal inflammatory response is detected. Cells stained with haematoxylin and eosin, (scale bars, 100 μm). The large region stained purple in the saline image is a hair follicle, while adipose tissue appears white in both images. Figure 4a shows the results of an assay that measures the haemolytic potential of adhesives that differ in their PEI content. The potential of the adhesive to lyse red blood cells increases slightly with PEI content, but in general, is very low. For adhesives composed of 6.9 wt% PEI or less, the percent haemolysis (~\n5%) is within the guidelines established by the ASTM (see protocol ASTM-F756). In our study, cells introduced to TCTP with and without added Triton-X served as controls. Figure 4b shows a suite of micrographs that correspond to the data shown in Fig. 4a . The images show erythrocytes resting on the TCTP control surface as well as the different adhesive surfaces. Cells display typical healthy round morphology, supporting the assertion that these surfaces are non-haemolytic. In contrast, when the detergent Triton-X is added, full haemolysis is evident. The cytocompatibility of the adhesive towards mammalian cells and tissue was further assessed in vivo . Figure 4c shows histological analysis of murine tissue obtained from regions of muscle, subcutaneous adipose tissue and dermis comprising the subcutaneous injection site. Separate subcutaneous injections of saline and a 6.9 wt% PEI adhesive were introduced to BALB/c mice, which were killed after 7 days. The left panel shows tissue from the saline sham and the right panel shows tissue from the adhesive injection. The two samples are nearly indistinguishable with the apparent absence of necrotic tissue or any foreign body reaction, indicating that the adhesive is conducive to cellular contact in a biological context. Figure 4: In vitro and in vivo biocompatibility of adhesive. ( a ) Haemolytic activity of adhesives as a function of PEI wt% along with the control TCTP surface with and without Triton-X (TX) ( n =3; error bars, s.d.). ( b ) Phase-contrast images of hRBCs plated on adhesives of varying PEI wt% or on the control TCTP surface with and without Triton-X (TX) (scale bars, 20 μm). ( c ) Histological examination of tissue at the injection site for the sham saline injection and the adhesive. No necrosis is evident in either sample and minimal inflammatory response is detected. Cells stained with haematoxylin and eosin, (scale bars, 100 μm). The large region stained purple in the saline image is a hair follicle, while adipose tissue appears white in both images. Full size image In vivo activity of bioadhesive hydrogel The in vivo antibacterial properties of the adhesive were assessed using two independent models of infection. The first model involves the direct injection of bacteria to the material implant site of mice. The second experiment uses a cecal ligation and puncture model of sepsis. In the first model, a single hydrogel formulation (2.5 wt% PDA cross-linked with 6.9 wt% PEI) was injected subcutaneously into BALB/c mice using a dual-barrel syringe after which a large number of bacteria, 10 8 CFU ml −1 S. pyogenes , were directly injected into the subcutaneous pocket where the hydrogel was injected to ensure bacteria/material contact. As a positive control for infection, the same concentration of S. pyogenes was injected subcutaneously into mice that did not contain the adhesive. When a clinically evident infection had developed in the control mice (~\n3 days), both control and experimental animals were killed and macroscopic images were taken at the injection site ( Fig. 5a ). For the S. pyogenes positive control, a large abscess can be visualized externally, which is not apparent in mice injected with the adhesive and bacteria, together. Internal examination of the abscess shows a significant amount of frank pus formation when the bacteria are injected alone. In comparison, when the bacteria were injected into the pocket that contained adhesive, normal skin morphology was observed with no apparent gross inflammation. Each site of injection was clinically scored according to infection grade, which operates on a scale of 0 to 4 based on the potential of swab samples, taken from the injection site, to establish colonies ex vivo on agar [32] . A score of 0 is given when swab samples are unable to produce colonies and indicated that the tissue, from which the swab was taken, harbour no bacteria. Conversely, scores of 1, 2, 3 or 4 indicated the quadrants in which bacteria establish colonies in a quadrant-streaked plate. Thus, a score of 4 indicates bacterial growth in all four quadrants and that the tissue site from which the swab originated was highly infected. 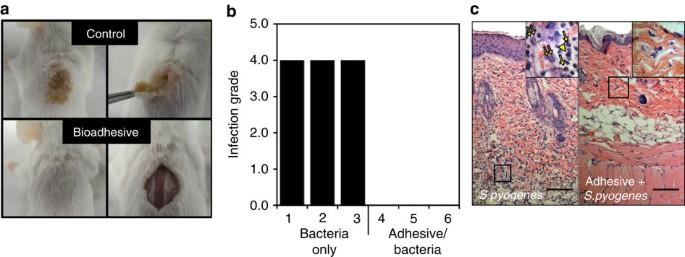Figure 5:In vivoassessment—with direct injection of bacteria. (a) Gross external (left) and internal (right) anatomical images of mice injected subcutaneously with 108CFU ml−1ofS. pyogenesdirectly into the back (control) or into adhesive (2.5 wt% PDA cross-linked with 6.9 wt% PEI) after 3 days (n=3). (b) Infection grade of primary tissue at injection site from mice injected with either bacteria only (control) or bacteria injected into adhesive. (c) Histological examination of the inflammatory response toS. pyogenes or adhesive injected withS. pyogenes. Cells stained with haematoxylin and eosin, (scale bars, 100 μm). Insets show × 100 magnification of the designated region. Inflammatory cells were identified based on cell morphology with →, ↔ and▸(in yellow) corresponding to neutrophils, macrophages and lymphocytes, respectively. Figure 5b shows the score results of the two groups of mice injected with S. pyogenes alone and S. pyogenes with the adhesive. In all cases where the adhesive was not present, mice developed a high-grade (4) infection. In contrast, bacteria directly injected into the adhesive resulted in a score of 0, indicating that the tissue site was free of viable bacteria. In an additional control experiment, bacteria were injected into mice at a site distal from a separate injection of the adhesive. This further tests our mechanistic understanding that bacteria must engage the adhesive to be killed. These control mice developed high-grade infections, suggesting that the mechanism of action for the adhesive may be contact-dependent ( Supplementary Fig. 3 ). Figure 5: In vivo assessment—with direct injection of bacteria. ( a ) Gross external (left) and internal (right) anatomical images of mice injected subcutaneously with 10 8 CFU ml −1 of S. pyogenes directly into the back (control) or into adhesive (2.5 wt% PDA cross-linked with 6.9 wt% PEI) after 3 days ( n =3). ( b ) Infection grade of primary tissue at injection site from mice injected with either bacteria only (control) or bacteria injected into adhesive. ( c ) Histological examination of the inflammatory response to S. pyogen es or adhesive injected with S. pyogen es. Cells stained with haematoxylin and eosin, (scale bars, 100 μm). Insets show × 100 magnification of the designated region. Inflammatory cells were identified based on cell morphology with →, ↔ and ▸ (in yellow) corresponding to neutrophils, macrophages and lymphocytes, respectively. Full size image Histology was performed to study the inflammatory response towards S. pyogenes in the absence and presence of the adhesive ( Fig. 5c ). Skin sections from mice exposed to S. pyogenes (left panel) or hydrogel and S. pyogenes (right panel) were stained with haematoxylin and eosin. A common inflammation scoring system was used with a range of 0 to 3 (ref. 33 ). Here a score of 0 indicates no or minimal infiltration of white blood cells into the injection area, whereas a score of 1, 2 or 3 denotes a single cell cluster, moderately diffuse or highly diffuse white blood cell invasion, respectively. A strong inflammatory response was observed for mice injected with S. pyogenes alone, resulting in a histological score of 3. In contrast, when S. pyogenes was administered at the site of bioadhesive injection, a weak inflammatory response was detected with a score of 1. As no active infection was detected, this weak immune response is most likely to be due to bacterial debris remaining from the action of the adhesive. This is consistent with the fact that when the bioadhesive was injected alone, minimal or no inflammation response was detected ( Fig. 4c ). In a second experiment, the gel was tested using a sepsis cecal ligation and puncture model [34] . Here, the ceca of mice were ligated and then punctured with a 20-gauge needle. If untreated, bacterial leakage from the intestine results in sepsis and death within 2–3 days. Application of the adhesive gel to the puncture area should form a barrier between the cecum and peritoneal cavity, and inhibit bacterial infiltration/translocation. 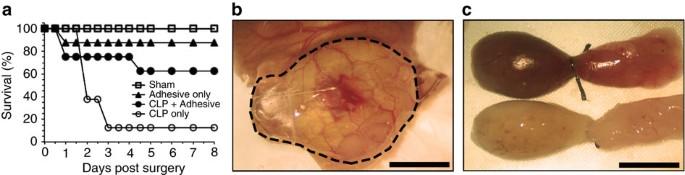Figure 6:In vivoassessment with a cecal ligation and puncture model. (a) Survival curves for sham, adhesive only, cecal ligation and puncture (CLP) with application of adhesive (2.5 wt% PDA cross-linked with 6.9 wt% PEI) and CLP only (n=8). (b) Application of adhesive to the punctured cecum during surgery (scale bar, 0.13 cm). Application area outlined. (c) Isolated punctured caeca 24 h after surgery. Control cecum (top) and experimental cecum that received gel (bottom) are shown (scale bar, 0.25 cm). Figure 6a contains survival curves that show that five out of eight mice treated with adhesive survived (63%) until the termination of the study at day 8. Only one mouse in the control group survived (13%) over this same time. The figure also shows that when gel is administered to animals without punctures, survival is high. This observation along with the fact that all animals recover weight loss ( Supplementary Fig. 4 ) after 4–5 days indicate that the gels are per se non-toxic. Figure 6b shows that when the adhesive is applied to the puncture area, a thin film forms over the resulting haematoma that seals the cecum. Figure 6c shows representative gross anatomical pictures of both control (top) and experimental (bottom) cecum isolated from animals 24 h after the start of the experiment. The control cecum to which a puncture was made but no adhesive administered is highly erythematous and appears dark in colour, indicating severe gross infection. In contrast, the experimental punctured cecum to which adhesive had been applied appears healthy and normal in colour, indicating that the gel had formed an effective barrier to infection. Figure 6: In vivo assessment with a cecal ligation and puncture model. ( a ) Survival curves for sham, adhesive only, cecal ligation and puncture (CLP) with application of adhesive (2.5 wt% PDA cross-linked with 6.9 wt% PEI) and CLP only ( n =8). ( b ) Application of adhesive to the punctured cecum during surgery (scale bar, 0.13 cm). Application area outlined. ( c ) Isolated punctured caeca 24 h after surgery. Control cecum (top) and experimental cecum that received gel (bottom) are shown (scale bar, 0.25 cm). Full size image Degradation of bioadhesive under physiological conditions Lastly, weight loss degradation studies were performed ex-vivo for the PDA–PEI adhesive gels showing that they degrade very slowly with over 60% of the adhesive remaining intact after 1 month ( Supplementary Fig. 5a ). These studies indicated that our gel degrades by bulk erosion as opposed to surface erosion [35] . In this biphasic mechanism, the material erodes at a defined erosion rate ( k deg ) until the network can no longer sustain the gelled state and undergoes immediate reverse gelation (a phase transition to the liquid state) that occurs at a definitive time ( t c =time to reverse gelation) [36] . The high RNH 2 /RCHO ratios (>1) used in the formulations result in substantial cross-linking and slow degradation rates, with k deg values (~\n0.07 per day) that are largely invariant over the time period assessed. As a result of the slow erosion rates, full degradation profiles were not feasible to collect in a reasonable time period and thus t c could not be experimentally determined for these formulations. We initially attempted to prepare gels with lower RNH 2 /RCHO ratios to observe t c in a reasonable time frame. However, formulations having low concentrations of PEI are not able to form competent gels. Thus, we developed a series of model gels where the PEI, an extremely amine-rich polymer, was replaced with BSA, a lysine-containing protein, as the cross-linking component of the gel. On a molecular basis, BSA has ~\n75% less solvent exposed amines compared with PEI that are available for cross-linking to the PDA component. These PDA–BSA formulations formed competent gels with RNH 2 /RCHO ratios <1, enabling t c to be measured in under 30 days ( Supplementary Fig. 5b ). Importantly, we found that t c is linearly dependent on the RNH 2 /RCHO ratio ( Supplementary Fig. 5c ), allowing values of t c to be extrapolated for the PDA–PEI gels. This assessment predicts t c times that vary from 10 to 30 months for the PDA–PEI gels ( Supplementary Fig. 5d ). Surgical site infections, especially at incision sites and in dead spaces, impair wound healing and, in extreme cases, lead to deep tissue necrosis and severe morbidity. Syringe-deliverable adhesives prepared from mixing solutions of PDA and branched PEI are mechanically stiff and provide adhesive strengths on par with fibrin glue. Importantly, these adhesives are inherently antibacterial, killing both Gram-negative and Gram-positive bacteria. Formulation studies indicate that the adhesive’s antibacterial activity is imparted by the electropositive charge afforded by the PEI component of the material. These studies further demonstrated that both the antibacterial action and the haemolytic potential of the adhesive material increases as the relative wt% of PEI in the formulation increases. However, an optimal adhesive prepared from 2.5 wt% oxidized dextran and 6.9 wt% PEI forms a potent antibacterial material, with good mechanical properties, that is minimally haemolytic. In vivo experiments show that this adhesive is potently effective in two independent murine models of infection, being able to kill bacteria while sparring mammalian host cells. Dynamic oscillatory rheology Oscillatory rheology experiments were performed on preformed adhesive gels using a TA Instruments’ AR-G2 rheometer, using an 8-mm diameter crosshatched stainless steel parallel plate tool. Hydrogels were prepared by first dissolving 5 mg of PDA (52% functionalized, M p =20.3 kDa, M n =15.5 kDa, M w / M n =1.4) in 100 μl of buffer (23.5 mM NaH 2 PO 4 , 80.6 mM Na 2 HPO 4 ) resulting in a 5 wt% solution. To this, an equal volume of 20.6 wt% PEI was added and a volume of 150 μl of the resulting mixture was quickly transferred to an empty well of a ProPlate Multi-Array Slide Module systems (P37001). The hydrogel was allowed to form for 10 min in an incubator set at 37 °C after which the resulting 2.5 wt% PDA, 10.3 wt% PEI hydrogel was removed from the well and cut to a height of ~\n2 mm with a scalpel. The other gel compositions were made in a similar fashion by adjusting the initial concentration of PEI. At any rate, hydrogels were individually transferred to a 25 °C pre-equilibrated rheometer and the tool lowered to a gap height of 1.9 mm (~\n5% strain). Standard S6 oil was placed around the tool to prevent evaporation during the measurements. For the gelation experiments, a short dynamic time sweep was performed to measure the storage (G′) and loss (G″) moduli at an angular frequency of 6 rad s −1 and 0.2% strain for 10 min to ensure the gel had equilibrated. A dynamic frequency sweep (0.1–100 rad s −1 , 0.2% strain) was then performed, where the average G′ was calculated from the value obtained at 6.3 rad s −1 (which is in the linear regime) from four independent measurements. Before performing these experiments, a dynamic strain sweep (0.1–1,000% strain, 6 rad s −1 ) on separate hydrogels were performed, and along with the frequency sweep data, ensured that G′ and G″ were measured in the linear regime ( Supplementary Fig. 6 ). Adhesive stress determination with porcine skin Porcine skin was purchased from Wagner’s meats (Mt. Airy, MD), any fat was removed from the dermal tissue layer and skin sections were cut to ~\n2 × 6 cm. The sectioned skin was soaked in PBS at 4 °C overnight and allowed to warm to room temperature (25 °C) before adhesive testing. A 75 μl mixture of 2.5 wt% PDA and 10.3 wt% PEI was applied between two tissue sections. The adhesion sample was incubated at 37 °C for 10 min with the application of ~\n100 g per sample to the exposed surface of the adhesive area. Samples were cooled to room temperature (25 °C) and adhesion stress was determined using a G2-RSA (TA Instruments) dynamic mechanical analyser. A tensile load was applied to the adhesive sample at a rate of 0.10 mm s −1 and the adhesive stress was monitored ( Supplementary Fig. 7 ). The maximum adhesive stress was considered to be the stress at which the two sample tissue sections became completely separated, concomitant with bond failure. The other gel compositions were assessed in a similar manner by adjusting the concentration of PEI. Bacteria culture and maintenance E. coli (25,922), S. aureus (25,923) and S. pyogenes (11,434) were purchased from ATCC and provided as a lyophilized powder. For all strains, the bacteria powder was suspended in 1 ml of tryptic soy broth (TSB) and subsequently quadrant streaked on a Trypticase soy agar plate containing 5% sheep blood. Bacteria were quadrant streaked daily and were used for experimentation once they had been streaked for 7 days on re-suspension. Material surface antibacterial properties Adhesive gels used for antibacterial assessment were prepared by adding an equal volume (50 μl) of PEI to 50 μl of a 5-wt% PDA solution (PDA, 52% functionalized, M p =20.3 kDa, M n =15.5 kDa, M w / M n =1.4). A volume of 70 μl of this mixture was immediately transferred to each well of a 96-well plate. The hydrogels were incubated at 37 °C for 30 min after which all hydrogels were washed to remove any un-cross-linked PEI and ensure the pH was equilibrated. First, the adhesive gels were rinsed with Dulbecco’s PBS (DPBS) three times, with the third wash allowed to incubate for 10 min at 37 °C. Next, the gel surfaces were washed with TSB three more times, with the second and third final wash allowed to incubate for 10 min at 37 °C. For all bacteria strains examined, a single colony of bacteria from the fourth quadrant of the agar growth plate was isolated and suspended in 1 ml of TSB. The optical density at 625 nm (OD 625 nm ) was adjusted to 0.1 AU by the addition of TSB, corresponding to a 10 8 CFU ml −1 stock bacteria solution. For the wt% PEI-dependent experiments, the stock was further diluted to 10 4 CFU ml −1 in TSB and 100 μl was introduced to the surface of the hydrogel or TCTP as a control. The bacteria were incubated on the hydrogel or TCTP surfaces for 24 h at 37 °C after which OD 625 nm of the solution above the gel was measured by the addition of 100 μl of bacteria-free TSB, followed by careful mixing and transfer to a cuvette to measure OD 625 nm . To determine the effect of the concentration of bacteria on the antibacterial properties of the adhesive surface, a volume of 90 μl bacteria-free TSB was introduced to the surface of freshly washed hydrogels, except for one. To the remaining hydrogel, 100 μl of the 10 8 CFU ml −1 bacteria stock solution was introduced. Subsequent 1:10 serial dilutions were performed down the plate by taking 10 μl of the bacterial suspension and adding it to the 90 μl of bacteria-free TSB in the adjacent well. As a control, bacteria were introduced to TCTP surfaces. To convert from CFU ml −1 to CFU dm −2 , the total CFUs was divided by the surface area of the gel or TCTP surface, which is dictated by the surface area of the well (0.0032, dm 2 ). Bacteria on control and adhesive surfaces were incubated for 24 h at 37 °C after which bacterial growth was assessed by measuring the OD 625 nm of the solution above the gel by the addition of 90 μl of bacteria-free TSB, gentle mixing and then transferring to a cuvette. Corrected OD 625 nm was calculated as follows: where the dilution factor is accounted for by the multiplication of 2 and: The Expected OD 1100, nm was calculated as follows: The is a constant that is specific to the strain of bacteria and is 3.19(.19), 3.21(0.13) and 2.80(0.14) for E. coli , S. aureus and S. pyogenes, respectively. Corrected OD 625 nm was converted to percent viability as follows: Contact-dependent antibacterial assessment Adhesive gels were prepared in transwell cell culture inserts at a volume of 350 μl. The hydrogel surfaces were washed by the addition of 700 μl of DPBS to the bottom of each well in a 24-well plate, and an additional 100 μl of DPBS was added to the top surface. The washes were repeated two additional times, with the third and final wash allowed to incubate at 37 °C for ~\n10–15 min. A 10 8 CFU ml −1 bacteria stock was prepared as indicated previously, and diluted to 10 4 CFU ml −1 with bacteria-free TSB. A volume of 500 μl of this solution was introduced to a given well and the freshly washed hydrogel contained in the transwell insert was positioned above the bacterial suspension. An additional 100 μl of bacteria-free TSB was supplemented to the top of the hydrogel to prevent evaporation. As a control, soluble PEI at the same concentration and volume was added to a transwell insert and incubated above the bacteria. In addition, untreated bacteria were included as a negative control. Sample plates were incubated at 37 °C for a total of 24 h, after which bacterial growth was assessed following the addition of 500 μl of TSB. Fluorescent imaging of bacteria on bioadhesive Mueller Hinton (MH) agar gels were prepared in six-well plates according to the manufacturer’s instructions. Briefly, 3.8 g of MH agar was dissolved in 100 ml of milli-Q water and then autoclaved for 15 min at 121 °C. After cooling to 50 °C in a water bath, a volume of ~\n1.5 ml of the agar solution was added to each well in a six-well plate and allowed to cool to room temperature for 30 min, resulting in an agar gel. A circular piece (9 mm in diameter) of the agar was removed by incision to reveal the underlying polystyrene. A 50-μl, 2.5 wt% PDA cross-linked with 6.9 wt% PEI gel, prepared as mentioned previously, was used to fill the cavity. The bioadhesive was incubated at 37 °C for 10 min, after which the gel surfaces were washed five times with 5 ml of PBS to remove any un-cross-linked PEI and ensure the pH was equilibrated. A volume of 500 μl of 10 8 CFU ml −1 of E. coli was added to each well and gently rocked to provide full surface coverage. As a control, E. coli was added to an MH agar gel void of bioadhesive. The plates were incubated for 24 h and then dyed with Syto9. Images were taken on a Zeiss AxioVert microscope. Percent haemolysis and hRBC imaging Adhesive gels were prepared and rinsed, with DPBS only, as indicated in the antibacterial hydrogel surface properties section. Human red blood cells (hRBCs) were isolated from blood samples provided by the Frederick Research Donor Program from healthy volunteers. The hRBCs were separated from the serum and washed three times with sterile DPBS by centrifugation at 3,460 r.p.m. for 10 min at 4 °C. Next, 30 μl of hRBCs were suspended in 12 ml of DPBS resulting in a 0.25% (v/v) cell suspension. Eighty microlitres of hRBCs were added to the surface of the hydrogels or a control TCTP surface. An additional 170 μl of DPBS was added to each well, resulting in a final solution of 0.08% (v/v) hRBC suspension. As a positive control, a 0.08% hRBC suspension was incubated with 0.2% Triton-X. The plate was incubated at 37 °C with agitation for 1 h after which 180 μl of the supernatant was transferred to an eppendorf tube and centrifuged at 14,000 r.p.m. at 4 °C for 10 min to remove any intact cells. Haemolytic activity was assessed by measuring the amount of haemoglobin liberated to the surrounding solution due to membrane rupture. The amount of haemoglobin released was determined by measuring the absorbance at 415 nm. Controls defining 0 and 100% haemolysis were hRBCs plated in DPBS on TCTP in the absence or presence of 0.2% Triton-X, respectively. For phase-contrast imaging, after the 1 h incubation the supernatant above the gels and TCTP were mixed gently by pipetting and 150 μl was transferred to an empty well of a 96-well plate. Images were collected on a Zeiss AxioVert microscope. Degradation studies Bioadhesive gel degradation was monitored by material weight loss as a function of time. Hydrogels, 200 μl in volume, were prepared in a ProPlate Multi-Array Slide Module system as previously mentioned and were incubated at 37 °C for 30 min before the onset of the degradation experiment. Next, preformed hydrogels were transferred to a cell separator where they were suspended in 10 ml of DPBS confined in a six-well plate. The plate was incubated at 37 °C with agitation (90 r.p.m.). At specified time points hydrogels were removed, gently blotted on a paper towel to remove any excess buffer, placed in a pre-weighed eppendorf tube and lyophilized. DPBS buffer, 10 ml, was replenished every 3 days. Time zero was considered to be a freshly prepared hydrogel directly placed in a pre-weighed eppendorf tube and lyophilized. PDA-BSA gels were prepared in the same manner, except that 7.5 wt% PDA was used and degradation assessed as for the PDA–PEI hydrogels. Degradation data is reported as percent weight loss versus time ( Supplementary Fig. 5 ). All gels degrade via bulk erosion that is characterized by an initial slow phase, defined by a single rate constant k deg , followed by a rapid reverse gel phase transition that occurs at time t c . The rate constant, k deg , was determined by fitting the initial slow phase of degradation using the fractional mass loss equation: M t / M o = k deg t n , where M t /M o is the fractional mass loss, t is time and n is the geometrical factor (0.5 for slabs). For the PDA–BSA gels, t c is the time at which <5% gel remains. As the PDA–PEI gels degrade very slowly, values of t c were determined by extrapolation using the linear relationship between the RNH 2 /RCHO ratio and t c as determined for the PDA–BSA gels ( Supplementary Fig. 5 ). Subcutaneous injection of bacteria All animal procedures were conducted in accordance with and after approval from Johns Hopkins Animal Care and Use Committee guidelines. Initially, ex-vivo antibacterial assays were performed using S. pyogenes similar to those shown in Fig. 2 to ensure that the adhesive was active toward this strain ( Supplementary Fig. 8 ). For the animal studies, five groups of 6- to 8-week-old BALB/c mice were used where each group contained two to three mice. Group one ( n =3) was injected with a sham injection of saline only subcutaneously above the dorsal thoracic midline. Group two ( n =3) was injected with ~\n100 μl bioadhesive gel (2.5 wt% PDA cross-linked with 6.9 wt% PEI) subcutaneously above the dorsal thoracic midline. Group three ( n =3) was injected with 70 μl of 10 8 CFU ml −1 S. pyogenes . Group four ( n =3) was injected with ~\n100 μl bioadhesive gel (2.5 wt% PDA cross-linked with 6.9 wt% PEI) subcutaneously above the dorsal thoracic midline followed by an injection of 10 8 CFU ml −1 S. pyogenes directly into the existing gel. Group five ( n =2) was injected with both 100 μl of bioadhesive followed an injection of 70 μl of 10 8 CFU ml −1 S. pyogenes at a distal site such that the bacteria did not come in contact with the gel. Groups 1 and 2 were killed at 7 days. Groups 3–5 were killed at 3 days when infection was apparent in the bacteria alone animals (Group 3). Infection grade was determined at the injection site by swabbing the site with a sterile cotton swab and streaking onto one quadrant of a 5% sheep blood agar plate. Subsequent quadrant streaking was performed for the remaining three quadrants using a new inoculating loop between each quadrant. The plates were incubated for 48 h at 37 ° C, after which colony formation was assessed. Infection grade was determined on a scale of 0, 1, 2, 3 or 4, based on the number of quadrants where colony formation was observed. Histology on the tissue sections from the injection site was performed to determine the immune response. After mice were killed, fresh tissue samples were obtained from the injection site, fixed in 10% normal buffer formalin and embedded in paraffin. Skin sections were cut to 5 μm and then stained with haematoxylin and eosin. Cecal ligation and puncture model Six- to eight-week-old male C57BL/6 mice were used for this experiment ( n =8 per group). Animals were anaesthetized with inhaled isoflurane and the abdomen was then shaved and disinfected by first applying betadine solution followed by wiping with a 70% alcohol swab. All procedures were performed under clean but not sterile conditions. A 1.5-cm midline laparotomy was performed to expose the cecum. Next, the cecal pole was tightly ligated with a 6.0 silk suture at 0.5 cm from its tip, and then perforated once with a 20-gauge needle. In the experimental group, the cecum was covered with the adhesive gel (2.5 wt% PDA cross-linked with 6.9 wt% PEI) before returning it back to the peritoneal cavity, whereas in the control group the cecum was directly returned to the peritoneal cavity. The abdominal wall was then closed in layers using a 6.0 silk running suture for the peritoneum and a 6.0 nylon suture for the skin. All animals were resuscitated by injecting 1 ml of pre-warmed 0.9% saline solution subscutaneously using a 25-guage needle. Buprenorphine (0.05 mg kg −1 ) was injected subcutaneously for postoperative analgesia. The animals were then placed on a heating pad until full recovery. Free access to food and water was ensured post surgery. Mice were monitored every 12 h for survival and weight loss. Lastly, calorimetric analysis, NMR characterization, and size exclusion chromatography analysis of the polydextran aldehyde used to formulate the bioadhesive is shown in Supplementary Figs. 9, 10 and 11 , respectively. How to cite this article: Giano, M. C. et al. Injectable bioadhesive hydrogels with innate antibacterial properties. Nat. Commun. 5:4095 doi: 10.1038/ncomms5095 (2014).